Versatilein vitrosystem to study translocation and functional integration of bacterial outer membrane proteins Gram-negative bacteria use the type-V secretion pathway to expose proteins at their cell surface, many of which have virulence functions. Translocation of those proteins across the outer membrane occurs either by means of dedicated translocator proteins (two-partner secretion) or covalently fused translocator domains (autotransporters). Translocator proteins and translocator domains are β-barrels requiring the β-barrel assembly machinery (BAM) for membrane integration. However, the molecular details of their passage across the envelope and insertion into the outer membrane remain enigmatic, owing in part to the fact that in vitro systems are not available. Here we describe a versatile in vitro reconstitution system that faithfully reproduces both branches of the type-V secretion pathway and the assembly of β-barrel outer membrane proteins. This system will allow an in-depth analysis of protein secretion across and integration into outer membranes. The inner and outer membranes of Gram-negative bacteria possess a number of individual as well as concerted machineries for the integration, translocation and secretion of newly synthesized proteins [1] , [2] , [3] . While protein transport events mediated by the Sec and Tat machineries of the inner membrane are reasonably well understood [3] , [4] , less is known about the mechanisms by which proteins cross or insert into the outer membrane. This lack of information is largely due to the scarcity of appropriate biochemical assays. The secretion of proteins across the outer membrane of Gram-negative bacteria occurs by at least eight different pathways, termed type-I–type-VIII secretion pathways. Among them, the type-V secretion pathway has attracted particular attention because it secretes clinically important virulence factors [5] and is potentially useful for secreting or displaying recombinant proteins [6] . Type-V secretion encompasses two major routes, the two-partner secretion (TPS) [7] and the autotransporter pathway [8] , [9] . As suggested by its name, TPS involves two proteins: a secreted TpsA protein and its cognate TpsB transporter in the outer membrane. Conversely, autotransporters are two domain proteins consisting of an amino-terminal secreted passenger domain and a carboxy-terminal domain, which was originally believed to be the sole requirement for the translocation of the passenger domain, hence the misleading label of ‘autotransporter’. One of the unique features of the outer membrane of Gram-negative bacteria—as well as those of mitochondria and chloroplasts—is its high content of β-barrel outer membrane proteins (OMPs) [10] , [11] , [12] , [13] , [14] , [15] . In bacteria, the biogenesis of β-barrel OMPs depends on the β-barrel assembly machinery (BAM), which in γ-proteobacteria is composed of five components, named BamA–E. The central BAM component, BamA, itself is a β-barrel protein that belongs to the Omp85 family [10] , [11] , [12] , [13] , [14] , [15] . Omp85 family members function in the intramembrane formation of β-barrels, while another group, represented by the above-mentioned TpsB proteins, facilitates translocation of the TpsA passenger proteins across the outer membrane. How β-barrel proteins of the Omp85 family can fulfil such seemingly diverse tasks such as protein translocation and formation of β-barrels has remained a matter of speculation. Recent X-ray crystal structures of BamA homologues revealed a lateral gate that may allow exit of a prefolded OMP or otherwise take part in the formation of a new β-barrel [16] , [17] , [18] . To enable a biochemical approach to these questions, we have developed a versatile cell-free system that allows the functional integration of Omp85 proteins into outer membrane-derived vesicles and thereby faithfully reproduces in vitro both the TPS and autotransporter pathways. This in vitro system therefore has the potential for an in-depth analysis of the OMP folding and assembly pathways. A cell-free system for monitoring OMP biogenesis We have devised an experimental system to study in vitro the transport of secreted proteins across, and the integration of β-barrel proteins into, the outer membrane of Gram-negative bacteria. In this system, we use spheroplasts of Escherichia coli (which lack an intact outer membrane) to express secreted and β-barrel membrane proteins. On induction and pulse labelling with [ 35 S]-methionine/cysteine, the target proteins are released from the Sec machinery into the surrounding medium of the spheroplasts, where they encounter proteoliposomes reconstituted with outer membrane translocation and integration factors. After removing the spheroplasts, the target proteins are then probed by various strategies for translocation and integration into the proteoliposomes. Translocation of TpsA proteins into TpsB proteoliposomes The 230-kDa filamentous hemagglutinin FhaB from Bordetella pertussis (TpsA protein) and its cognate outer membrane transporter FhaC (TpsB protein) constitute a typical TPS system. We recently achieved the translocation of a small N-terminal truncate of FhaB into FhaC-containing vesicles [19] . We now constructed a longer N-terminal fragment of FhaB about 60 kDa in size ( Fig. 1a , named FhaB*60). FhaB*60 was specifically expressed, pulse labelled and secreted from spheroplasts ( Fig. 1a , compare lanes 1 and 2). When FhaB*60 was secreted in the presence of proteoliposomes that had been reconstituted from total OMPs of an FhaC-expressing E. coli strain (OMP-PL+FhaC), about 30% of it became resistant towards digestion by proteinase K (PK; lanes 8 and 9). No PK-resistant FhaB*60 was, however, obtained when the membrane vesicles were disrupted by 1% Triton X-100 (lane 10). These findings are consistent with a complete translocation of FhaB*60 into the FhaC-containing OMP proteoliposomes. Translocation of FhaB*60 strictly required FhaC because it was virtually completely degraded by PK when FhaC-lacking OMP proteoliposomes (OMP-PL−FhaC, lanes 6 and 7) were used. The same was the case in the absence of any vesicles or in the presence of protein-free liposomes (lanes 2–5). To confirm that transport of FhaB*60 was truly dependent on a functional FhaC, various FhaC variants shown to affect FhaB translocation under in vivo conditions [16] , [20] were also tested. As depicted in Fig. 1a , lanes 11–16, translocation of FhaB*60 into proteoliposomes containing those FhaC mutants was indeed drastically reduced. Because equivalent amounts of wild-type and mutant FhaC species (except for ΔPOTRA1, in which case twice the amount of outer membranes compared with the ΔLoop6 mutant was used for solubilization and reconstitution) had been reconstituted into the proteoliposomes used for these assays ( Fig. 1b ), the impairment of translocating FhaB*60 ( Fig. 1a , lanes 8–16) can only be ascribed to the functional defects of the FhaC variants. Finally as shown in Fig. 1a (lanes 17 and 18), translocation of FhaB*60 was solely dependent on FhaC because translocation-proficient proteoliposomes were also obtained when reconstituted with purified FhaC only (see, for example, Fig. 1d , lane 9). 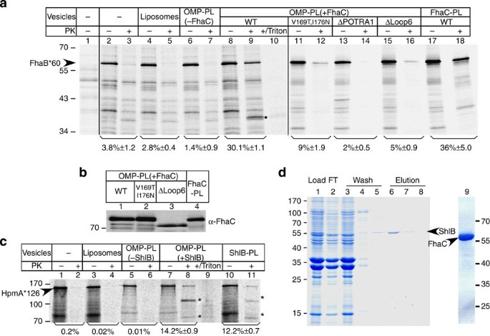Figure 1:In vitroreconstruction of TPS using various TpsA proteins. (a) Translocation of a 60-kDa N-terminal fragment ofB. pertussisfilamentous hemagglutinin (FhaB*60) into FhaC-containing proteoliposomes (PL). OMPs ofE. colicells deficient of FhaC or overexpressing wild-type FhaC or any of the indicated FhaC mutants were solubilized with Elugent and then reconstituted into proteoliposomes (OMP-PL−/+FhaC). In addition, purified FhaC (see, for example, paneld) was also reconstituted (FhaC-PL). FhaB*60 was expressed in spheroplasts, pulse-labelled with [35S]methionine/cysteine and incubated for 15 min at 37 °C in the presence of vesicles as indicated. After removing spheroplasts by low-speed centrifugation, supernatants were divided into two halves, one of which was treated with PK. After precipitation with TCA, the samples were run on 10% SDS–polyacrylamide gels and visualized by phosphorimaging. In lane 9, PK treatment was performed in the presence of 1% Triton X-100. The band labelled with a black dot might be a potential translocation intermediate. (b) Western blot analysis of the indicated FhaC variants-containing proteoliposomes using anti-FhaC antibodies. (c) Translocation of a 126-kDa N-terminal fragment ofP. mirabilisHpmA (HpmA*126) into proteoliposomes (PL) containing ShlB ofS. marcescens. In lanes 10 and 11, proteoliposomes were prepared from purified ShlB (ShlB-PL). Asterisks indicate uncharacterized degradation products of HpmA after PK treatment. (d) Purification of ShlB and FhaC via nickel affinity chromatography. Proteins were separated by SDS–PAGE and stained with Coomassie Blue. FT, flow through. Relative translocation efficiencies are the means (±s.d.) of three independent experiments. Figure 1: In vitro reconstruction of TPS using various TpsA proteins. ( a ) Translocation of a 60-kDa N-terminal fragment of B. pertussis filamentous hemagglutinin (FhaB*60) into FhaC-containing proteoliposomes (PL). OMPs of E. coli cells deficient of FhaC or overexpressing wild-type FhaC or any of the indicated FhaC mutants were solubilized with Elugent and then reconstituted into proteoliposomes (OMP-PL−/+FhaC). In addition, purified FhaC (see, for example, panel d ) was also reconstituted (FhaC-PL). FhaB*60 was expressed in spheroplasts, pulse-labelled with [ 35 S]methionine/cysteine and incubated for 15 min at 37 °C in the presence of vesicles as indicated. After removing spheroplasts by low-speed centrifugation, supernatants were divided into two halves, one of which was treated with PK. After precipitation with TCA, the samples were run on 10% SDS–polyacrylamide gels and visualized by phosphorimaging. In lane 9, PK treatment was performed in the presence of 1% Triton X-100. The band labelled with a black dot might be a potential translocation intermediate. ( b ) Western blot analysis of the indicated FhaC variants-containing proteoliposomes using anti-FhaC antibodies. ( c ) Translocation of a 126-kDa N-terminal fragment of P. mirabilis HpmA (HpmA*126) into proteoliposomes (PL) containing ShlB of S. marcescens . In lanes 10 and 11, proteoliposomes were prepared from purified ShlB (ShlB-PL). Asterisks indicate uncharacterized degradation products of HpmA after PK treatment. ( d ) Purification of ShlB and FhaC via nickel affinity chromatography. Proteins were separated by SDS–PAGE and stained with Coomassie Blue. FT, flow through. Relative translocation efficiencies are the means (±s.d.) of three independent experiments. Full size image We then tested an even longer TpsA passenger protein (HpmA*126) in combination with a heterologous yet complementary TpsB transporter (ShlB) [21] , [22] . HpmA is a 160-kDa hemolysin from Proteus mirabilis , of which we expressed a 126-kDa N-terminal fragment (HpmA*126) in spheroplasts. The TpsB translocator protein ShlB from Serratia marcescens was overexpressed in E. coli and reconstituted into proteoliposomes together with the pool of E. coli OMPs. As shown in Fig. 1c , HpmA*126 was degraded by PK when it was secreted from spheroplasts in the absence of membranes ( Fig. 1c , lanes 1 and 2) or in the presence of protein-free liposomes ( Fig. 1c , lanes 3 and 4). In contrast, secretion in the presence of ShlB-containing OMP proteoliposomes gave rise to three PK-resistant species ( Fig. 1c , lane 8), one corresponding in size to HpmA*126 and two smaller ones (asterisks), the nature of which has not been pursued any further. Resistance of the full-size HpmA*126 species against PK treatment was abolished in the presence of 1% Triton X-100 ( Fig. 1c , lane 9) indicating successful translocation into a proteoliposome-protected space. The translocation activity was dependent on ShlB, because OMP proteoliposomes lacking ShlB did not yield any PK-resistant HpmA*126 ( Fig. 1c , lanes 5 and 6). Furthermore, when the ShlB protein was purified from the pool of detergent-solubilized OMPs ( Fig. 1d ) and individually reconstituted into ShlB-proteoliposomes, it fully sustained translocation of HpmA*126 ( Fig. 1c , lanes 10 and 11). This emphasizes our previous conclusion that TpsB proteins (that is, ShlB and FhaC) are the sole translocators of TpsA passenger proteins [19] . In vitro reconstruction of autotransporter translocation The versatility of this experimental set-up was further tested using the autotransporter system of the bacterial outer membrane. Many autotransporters are large proteins composed of an N-terminal passenger domain being secreted and a C-terminal β-barrel domain that is integrated into the outer membrane and thereby enable secretion of the passenger domain. The denomination ‘autotransporter’ originally implied that the β-barrel domain would be sufficient to translocate the upstream passenger domain, whereas recent findings suggested that the autotransport process crucially depends on the BAM machinery [23] , [24] , [25] , [26] , [27] . The autotransporter we used was antigen 43 (Ag43) of E. coli , a surface protein that mediates cellular autoaggregation [28] . Like many monomeric autotransporters, Ag43 undergoes autoproteolytic processing between its N-terminal passenger domain (α 43 ) and its C-terminal β-barrel domain (β 43 ) (ref. 29 ). In fact, when Ag43 was produced by spheroplasts, a substantial amount of it was cleaved into two fragments that comigrated on SDS–polyacrylamide gel electrophoresis (PAGE) with the individually expressed α 43 - and β 43 -domains ( Fig. 2a , lanes 1–3). Since cleavage of Ag43 occurs between Asp551 and Pro552 [29] , we mutated Asp551 to Asn and Ala. Both mutations were found to block autoproteolysis as shown for the Ag43(D551N) variant in Fig. 2a (compare lanes 2 and 4). When Ag43(D551N) was treated with PK after its secretion from spheroplasts, an inherently PK-resistant product of around 74 kDa was obtained ( Fig. 2a , lane 5, *). In contrast, when secretion of Ag43(D551N) proceeded in the presence of OMP-containing proteoliposomes, the subsequent PK treatment gave rise to an additional resistant fragment of about 103 kDa ( Fig. 2a , lane 9). This membrane-protected fragment (MPF) was not obtained when OMP proteoliposomes were replaced by protein-free liposomes ( Fig. 2a , lanes 6 and 7), nor was it generated when the protease digestion was performed in the presence of 1% Triton X-100 to disrupt the OMP proteoliposomes ( Fig. 2a , lane 10), suggesting that the MPF was derived from an incomplete protection of Ag43(D551N) after its transport into OMP-containing proteoliposomes. 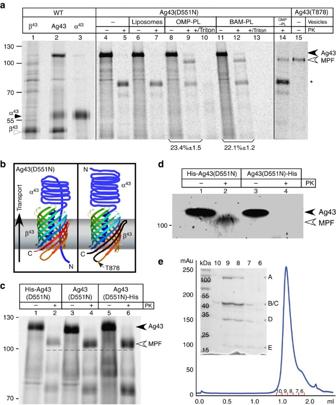Figure 2:In vitroreconstruction of autotransporter translocation. (a) Wild-type (WT) Ag43 and the individual α and β domains of Ag43 were overexpressed in spheroplasts and separated by 8% SDS–polyacrylamide gels. A substantial amount of Ag43 undergoes autoproteolysis (lane 2), which can be prevented by mutating Asp551 to Asn (Ag43(D551N)) (lane 4). Translocation experiments of Ag43(D551N) using OMP-PL (lanes 8 and 9) yield a MPF, which disappears by disrupting the OMP-PL with Triton X-100 (lane 10). Proteoliposomes reconstituted with purified BamA–E (BAM-PL) gave rise to the same MPF (lanes 11–13). The MPF comigrates with a C-termial truncate Ag43(T878) constructed on the supposition that PK might cleave Ag43(D551N) around residue T878. Asterisk represents an inherent PK-resistant product of Ag43(D551N). Relative translocation efficiencies are the means of three independent experiments. (b) Two possible configurations of Ag43(D551N) within membranes could lead to the formation of the MPF on PK treatment. The C-terminal fragment that is presumably removed during PK treatment is marked in black (right panel). (c) Two derivatives of Ag43(D551N) carrying 6 × histidine tags either at the N terminus (His-Ag43(D551N)) or C terminus (Ag43(D551N)-His) give rise to a slight band shift on 6% SDS–polyacrylamide gels (lanes 1 and 5) when compared with untagged Ag43(D551N) (lane 3). Following translocation of both derivatives into OMP-PL and PK treatment, the band shift of the MPF was retained only for His-Ag43(D551N) (compare lanes 2 and 6 with respect to the dashed line). (d) Proteins derived from 20-times scaled-up, non-radioactive reactions were resolved by SDS–PAGE (10% gels) and subjected to InVision His-tag in-gel staining. While the N-terminal His-tag is detectable suggesting complete sequestration by OMP-PL, the C-terminal His-tag is removed on PK treatment suggesting its exposure on the surface of OMP-PL. (e) BamA–E subunits were co-expressed inE. coliand purified from DDM-solubilized membranes using a Strep-Tactin affinity column followed by size-exclusion chromatography (SEC). Shown are a SEC chromatogram and a Commassie Blue-stained SDS gel of the indicated elution fractions. Figure 2: In vitro reconstruction of autotransporter translocation. ( a ) Wild-type (WT) Ag43 and the individual α and β domains of Ag43 were overexpressed in spheroplasts and separated by 8% SDS–polyacrylamide gels. A substantial amount of Ag43 undergoes autoproteolysis (lane 2), which can be prevented by mutating Asp551 to Asn (Ag43(D551N)) (lane 4). Translocation experiments of Ag43(D551N) using OMP-PL (lanes 8 and 9) yield a MPF, which disappears by disrupting the OMP-PL with Triton X-100 (lane 10). Proteoliposomes reconstituted with purified BamA–E (BAM-PL) gave rise to the same MPF (lanes 11–13). The MPF comigrates with a C-termial truncate Ag43(T878) constructed on the supposition that PK might cleave Ag43(D551N) around residue T878. Asterisk represents an inherent PK-resistant product of Ag43(D551N). Relative translocation efficiencies are the means of three independent experiments. ( b ) Two possible configurations of Ag43(D551N) within membranes could lead to the formation of the MPF on PK treatment. The C-terminal fragment that is presumably removed during PK treatment is marked in black (right panel). ( c ) Two derivatives of Ag43(D551N) carrying 6 × histidine tags either at the N terminus (His-Ag43(D551N)) or C terminus (Ag43(D551N)-His) give rise to a slight band shift on 6% SDS–polyacrylamide gels (lanes 1 and 5) when compared with untagged Ag43(D551N) (lane 3). Following translocation of both derivatives into OMP-PL and PK treatment, the band shift of the MPF was retained only for His-Ag43(D551N) (compare lanes 2 and 6 with respect to the dashed line). ( d ) Proteins derived from 20-times scaled-up, non-radioactive reactions were resolved by SDS–PAGE (10% gels) and subjected to InVision His-tag in-gel staining. While the N-terminal His-tag is detectable suggesting complete sequestration by OMP-PL, the C-terminal His-tag is removed on PK treatment suggesting its exposure on the surface of OMP-PL. ( e ) BamA–E subunits were co-expressed in E. coli and purified from DDM-solubilized membranes using a Strep-Tactin affinity column followed by size-exclusion chromatography (SEC). Shown are a SEC chromatogram and a Commassie Blue-stained SDS gel of the indicated elution fractions. Full size image We considered two possibilities for the partial cleavage of Ag43(D551N) by PK (see, for example, Fig. 2b ): it was due to either an incomplete transfer of the α 43 -domain across the membrane rendering its N terminus partially accessible to PK or the C terminus of the β 43 -domain of Ag43(D551N) remained partially exposed on the outside of the vesicles. To distinguish between the two possibilities, two derivatives of Ag43(D551N) were generated carrying a tag of six histidine residues either at the N terminus (His-Ag43(D551N)) or C terminus (Ag43(D551N)-His). When expressed in spheroplasts, both extended variants displayed a slightly reduced electrophoretic mobility on 6% SDS–polyacrylamide gels when compared with the untagged Ag43(D551N) version ( Fig. 2c , compare lanes 1 and 5 with 3). After exposure to OMP proteoliposomes and subsequent PK treatment only the MPF derived from the N-terminally His-tagged Ag43(D551N) retained the mobility shift (compare MPF in lanes 2 and 4), whereas that of the Ag43(D551N) variant carrying the C-terminal His-tag did not (MPF, lanes 4 and 6). These results indicate that the N terminus of Ag43(D551N) must have been completely translocated into the lumen of the OMP proteoliposomes, while the His-tagged C terminus obviously was cleaved off by PK on the outer surface of OMP proteoliposomes. To confirm these results, in-gel detection of the 6 × His-tags was performed after translocating the His-Ag43(D551N) and Ag43(D551N)-His variants into proteoliposomes using 20-times scaled-up translocation assays. As shown in Fig. 2d , only the N-terminal His-tag remained detectable after PK treatment (lanes 2 and 4). Altogether, these data demonstrate that after a full translocation of its α 43 -domain into the OMP proteoliposomes, Ag43(D551N) adopts a topology as depicted in Fig. 2b (right panel), in which the β 43 -domain is embedded within the membrane of OMP proteoliposomes with its C terminus being exposed on the surface of the vesicles. To map the presumed PK cleavage site in the β 43 -domain, we tried to determine the precise molecular size of the MPF of Ag43(D551N). By relating the apparent electrophoretic mobility of Ag43(D551N) (116.06 kDa) to its theoretical molecular size (101.2 kDa), the theoretical value of the size of the MPF (103.05) was calculated as 89.855 kDa. This would correspond to a predicted PK cleavage site between Thr878 and Phe879 located within a PK-accessible periplasmic loop of β 43 (according to PRED-TMBB) [30] . To verify this prediction, we mutated Thr878 of Ag43(D551N) to a stop codon-constructing Ag43(T878), expressed this truncate in spheroplasts and loaded the secreted material on SDS–PAGE for a direct comparison with the MPF. As shown in Fig. 2a (compare lanes 9 and 14 with 15), Ag43(T878) indeed runs at the same height as the MPF on SDS–PAGE, indicating that the formation of the MPF of Ag43(D551N) results from the cleavage within a periplasmic loop of the membrane-embedded β-domain as illustrated in Fig. 2b (right panel). Because a knockout of bamA interferes with autotransporter translocation in S. flexneri [23] and components of the BAM complex were found in close proximity to an autotransporter being assembled at the outer membrane of E. coli [26] , [27] , we tested if translocation of Ag43(D551N) into proteoliposomes could also be achieved if we replaced the total OMPs by the purified BAM components of E. coli only. As can be seen in Fig. 2a (lanes 11–13), proteoliposomes that had been reconstituted with the purified BamA–E proteins ( Fig. 2e ) in fact yielded the MPF indicative of translocation of the Ag43(D551N) passenger domain into the vesicles. Collectively, these data strongly suggest that the translocation process of an autotransporter was successfully reproduced in vitro and they also provide the first biochemical evidence that the BAM complex is functionally involved in the translocation of autotransporters. Functional integration of bacterial β-barrel OMPs in vitro We further exploited our experimental set-up for the BAM-dependent integration of β-barrel OMPs. Like most other proteins, β-barrel OMPs become completely denatured on boiling in SDS. However, they diagnostically retain a compact structure when treated with SDS only at moderate temperatures, resulting in a faster migration on polyacrylamide gels than the heat-treated control samples [31] , [32] . This so-called heat modifiability is demonstrated in Fig. 3 (lanes 1 and 2) for the β-barrel protein BamA recovered from E. coli outer membranes. 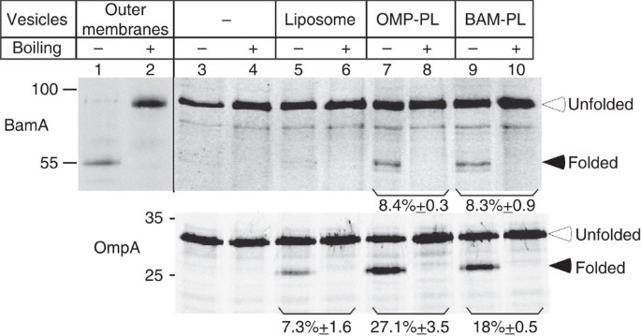Figure 3:In vitrointegration of bacterial β-barrel OMPs. BamA maintains a folded structure after SDS denaturation at room temperature. Outer membranes ofE. colistrain BL21(DE3) were subjected to electrophoresis under semi-native conditions and probed with α-BamA antibodies (lanes 1 and 2). Lanes 3–10, the OMPs BamA and OmpA were expressed, radioactively labelled and secreted fromE. colispheroplasts and subsequently integrated into membrane vesicles. Folded forms of BamA and OmpA suggesting their successful integrationin vitroare obtained in the presence of proteoliposomes containing OMPs and purified BamA–E proteins. Relative integration efficiencies are the means (±s.d.) of three independent experiments. Figure 3: In vitro integration of bacterial β-barrel OMPs. BamA maintains a folded structure after SDS denaturation at room temperature. Outer membranes of E. coli strain BL21(DE3) were subjected to electrophoresis under semi-native conditions and probed with α-BamA antibodies (lanes 1 and 2). Lanes 3–10, the OMPs BamA and OmpA were expressed, radioactively labelled and secreted from E. coli spheroplasts and subsequently integrated into membrane vesicles. Folded forms of BamA and OmpA suggesting their successful integration in vitro are obtained in the presence of proteoliposomes containing OMPs and purified BamA–E proteins. Relative integration efficiencies are the means (±s.d.) of three independent experiments. Full size image To test integration of β-barrel proteins into outer membrane-derived vesicles, the 35-kDa OmpA and the 95-kDa BamA were expressed, pulse-labelled and secreted from spheroplasts. Outer membrane-derived vesicles were reconstituted from phospholipids and detergent-extracted E. coli OMPs including the BAM complex that would be required for the integration of OmpA and BamA. The presence of BamA in these reconstituted proteoliposomes was verified using anti-BamA antibodies (see, for example, Fig. 4 ). After secreting the radiolabelled test OMPs, OmpA or BamA, spheroplasts were removed by centrifugation and the separated supernatants were incubated for 15 min with the OMP proteoliposomes to allow integration to occur. The mixture was then treated with SDS either at low temperature or 95 °C. In the absence of any membranes as well as in the presence of plain liposomes, spheroplast-secreted radiolabelled BamA virtually did not show heat modifiability ( Fig. 3 , lanes 3–6). The same results were obtained for OmpA, except that some folding was observed in the presence of plain liposomes ( Fig. 3 , lanes 5 and 6). The latter could be due to a lipid-induced spontaneous folding as previously demonstrated [33] , [34] . In contrast, when secreted in the presence of OMP-containing proteoliposomes ( Fig. 3 , lanes 7 and 8; OMP-PL), a fraction of both BamA and OmpA displayed a faster electrophoretic mobility indicative of the folded species that resisted SDS treatment at low temperature. These data are consistent with the integration and concomitant folding of the two test OMPs into the outer membrane-derived vesicles. The same results were obtained using proteoliposomes prepared from purified BamA–E proteins ( Fig. 3 , lanes 9 and 10; BAM-PL) indicating that in our system, the assembly of BamA and OmpA into heat-sensitive β-barrel structures was mediated by the function of the BAM complex. 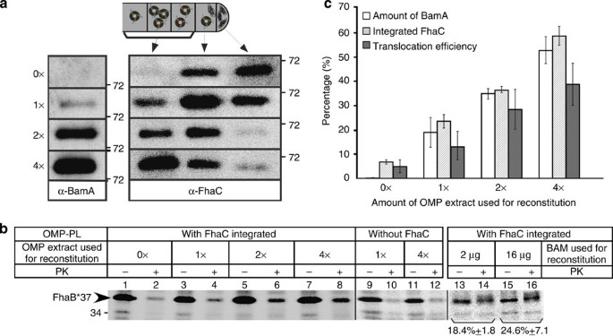Figure 4:In vitrointegrated FhaC is functional. (a) Reconstitution of proteoliposomes containing increasing amounts of OMPs (1 × , 2 × , 4 × ) as indicated by western blotting using α-BamA antibodies (α-BamA). These OMP-PL were used to integrate spheroplast-secreted, non-radioactively labelled FhaC. Thereafter, proteoliposomes were recovered by flotation centrifugation and analysed for their FhaC content by immunoblotting against anti-FhaC antibodies (α-FhaC). (b) FhaC-containing OMP- or BAM-PL were directly used to measure translocation of spheroplast-secreted radioactively labelled FhaB*37. (c) Quantification (s.d.) of the results derived froma,bas obtained from three independent experiments each. The relative amounts of BamA refer to that of proteoliposomes reconstituted from 8 × OMP extract. The percentage of the integrated FhaC is the sum of FhaC recovered from the top three fractions of each flotation experiment shown inarelative to the total amount of FhaC present in all five fractions. The translocation efficiency of FhaB*37 was calculated by quantifying the amount of PK-resistant FhaB*37 relative to that of each non-treated FhaB*37 species. Figure 4: In vitro integrated FhaC is functional. ( a ) Reconstitution of proteoliposomes containing increasing amounts of OMPs (1 × , 2 × , 4 × ) as indicated by western blotting using α-BamA antibodies (α-BamA). These OMP-PL were used to integrate spheroplast-secreted, non-radioactively labelled FhaC. Thereafter, proteoliposomes were recovered by flotation centrifugation and analysed for their FhaC content by immunoblotting against anti-FhaC antibodies (α-FhaC). ( b ) FhaC-containing OMP- or BAM-PL were directly used to measure translocation of spheroplast-secreted radioactively labelled FhaB*37. ( c ) Quantification (s.d.) of the results derived from a , b as obtained from three independent experiments each. The relative amounts of BamA refer to that of proteoliposomes reconstituted from 8 × OMP extract. The percentage of the integrated FhaC is the sum of FhaC recovered from the top three fractions of each flotation experiment shown in a relative to the total amount of FhaC present in all five fractions. The translocation efficiency of FhaB*37 was calculated by quantifying the amount of PK-resistant FhaB*37 relative to that of each non-treated FhaB*37 species. Full size image We then exploited the FhaB*37/FhaC TPS system [19] to demonstrate functionality of the BAM-dependent integration of a β-barrel protein in this in vitro system. To this end, we varied the amount of OMPs reconstituted into proteoliposomes on the premise that proteoliposomes containing increasing amounts of the BAM components should allow correspondingly more integration of the β-barrel translocator FhaC and this in turn enhances translocation of FhaB*37. An immunoblot developed with anti-BamA antibodies of OMP proteoliposomes that had been reconstituted with increasing amounts of outer membrane extract demonstrates the expected increase in the amount of reconstituted BAM machinery ( Fig. 4a , α-BamA, 1 × , 2 × , 4 × and the OMP-free control 0 × ). When these different vesicles were incubated with spheroplasts producing non-radioactively labelled FhaC and then freed from non-integrated FhaC by flotation centrifugation ( Fig. 4a , top), they in fact revealed a BamA-dependent increase in the amount of newly integrated FhaC ( Fig. 4a , α-FhaC; see also quantitation of three parallel experiments in Fig. 4c ). OMP proteoliposomes containing increasing amounts of integrated FhaC were then assayed for translocation of FhaB*37 ( Fig. 4b ). The obtained translocation efficiencies fully correlated with the amounts of in vitro integrated FhaC and reconstituted BamA ( Fig. 4c ). Proteoliposomes that had not been exposed to FhaC-producing spheroplasts showed only background translocation of FhaB*37 that was independent of their BamA content ( Fig. 4b , lanes 9–12). As a further confirmation for the BAM-mediated integration of FhaC, purified BamA–E proteins were used to prepare BAM proteoliposomes for repeating the above experiments and as expected, the same results were obtained ( Fig. 4b , lanes 13–16). Hence, the β-barrel protein FhaC had de novo integrated into proteoliposomes by the reconstituted BAM components, thereby endowing these vesicles with the capability to translocate FhaC’s cognate passenger protein FhaB*37. We have developed a cell-free system that faithfully reproduces the BAM-mediated membrane integration of Omp85 paralogues (FhaC and BamA) as well as other β-barrel proteins (OmpA and β 43 of autotransporter Ag43). A similar experimental strategy had previously been employed to unravel the sorting of lipoproteins to the outer membrane of E. coli [35] . Using our system, we were able to functionally reconstitute in vitro both branches of the type-V secretion route, TPS and autotransporter pathway. TpsA proteins of up to 120 kDa were completely translocated into TpsB-containing proteoliposomes and the previously reported transcomplementation between the non-cognate TpsA–TpsB pair, HpmA and ShlB [21] , [22] could also be established for our in vitro conditions. Using purified ShlB reconstituted into proteoliposomes, we could confirm our previous observation [19] that TpsB proteins represent the sole requirement for the translocation of TpsA proteins. This indicates that TpsB-type Omp85 β-barrel proteins operate as true and autonomous translocators. By reconstituting the purified BamA–E complex into liposomes, we obtained the complete sequestration of the passenger domain α 43 of the E. coli autotransporter Ag43 into the vesicle lumen. On the basis of the reasonable assumption that α 43 would not have been fully translocated without the downstream β-domain of Ag43 having been assembled in the lipid bilayer, we conclude that our results demonstrate the direct involvement of BAM in autotransporter biogenesis. Such an involvement had thus far only been deduced from the findings that stalled translocation intermediates of autotransporters associate with BAM subunits [24] , [26] , [27] and that depletion of BAM components from whole cells interferes with the secretion of various autotransporters [23] , [25] . Recently, a new ‘translocation and assembly module’ (TAM) was described, the depletion of which negatively affected the secretion of proteobacterial autotransporters such as Ag43 [36] . TAM consists of the OMP TamA, which is an Omp85 family member [37] , and the inner membrane protein TamB. Although we cannot entirely rule out traces of the Tam components contaminating our in vitro system, our data rather suggest that at least in vitro the assembly of Ag43 can be achieved solely by the BAM complex. Although spontaneous folding of purified β-barrel OMPs into lipid bilayers has been observed [33] , [34] , efficient integration in vivo depends on the essential function of Omp85 proteins [38] , [39] . Hagan et al . [40] recently demonstrated the successful refolding of a urea-denatured β-barrel protein by the isolated BamA–E complex of E. coli reconstituted into liposomes. In contrast, the in vitro approach that we describe here allows the de novo insertion and functional assembly of β-barrel proteins, thereby recapitulating the in vivo biogenesis of newly synthesized OMPs. Thus far, we obtained highest transport efficiencies by adding outer membrane-derived proteoliposomes directly to the spheroplasts synthesizing the secreted and β-barrel proteins. This would suggest that any delay between secretion across the plasma membrane of spheroplasts and targeting to the outer membrane might require the involvement of chaperones to keep substrate proteins’ transport competent. Our experimental set-up should now provide the basis for the identification of such chaperones. It should also prove very useful in elucidating the individual functional roles of the BamA–E components during the biogenesis of OMPs and it will be amenable to addressing questions of the energy sources required for type-V secretion and the precise role the TAM complex plays in the assembly of autotransporters. Plasmids FhaB*37 was expressed from plasmid pTrc99a::FhaB45met-His [19] . FhaC was expressed from plasmid pFJD118 [41] when used for the preparation of FhaC-containing proteoliposomes or for FhaC purification, and from pTrc99a::FhaC if it was to be secreted from spheroplasts. Plasmid pTrc99a::FhaC was constructed by cutting out the fhaC sequence from pFJD118 using the restriction enzymes XbaI/HindIII. This fragment was then ligated into pTrc99a digested with XbaI/HindIII. Plasmids encoding FhaC variants, in which either POTRA domain 1 (pAS01) or loop L6 (pAS03) were deleted or which carried the double mutations V169T and I176N (pFJD138), have been described [16] , [20] . ShlB was expressed from pAP561, which was a direct ligation product from a PCR amplification of pAP531 using the primers AJ1 and AJ2 ( Supplementary Table 1 ), while pAP531 is constructed in the same way by ligating the PCR amplification product of pAP501 [42] using the primers AJ3 and AJ4. OmpA was expressed from pTompA (pTrc99a::OmpA) [43] . Plasmid pTrc99a::FhaB*60 was constructed to encode an N-terminal ~60-kDa fragment of B. pertussis FhaB. The desired region was amplified from plasmid pFJD12 (ref. 44 ) using the primers DR1 and DR2. The resulting PCR product was digested with XhoI/BlpI, then ligated into pTrc99a digested with XhoI/BlpI. The HpmA*126-coding sequence of pFJD20 [22] was amplified using the phosphorylated primers DR3 and DR4 and the Q5 High-Fidelity PCR Kit (New England Biolabs). The resulting blunt-ended hpmA*126 PCR fragment was ligated directly into a pTrc99a derivative encoding an OmpA signal peptide, which was obtained from pTrc99a::FhaB45met-His by digestion with HindIII, blunt-end formation with the large Klenow fragment and dephosphorylation. In the final construct pTrc99a::OmpA sp /HpmA*126, the native signal peptide of HpmA is replaced with that of OmpA. The flu gene coding for Ag43 was amplified from chromosomal DNA of the E. coli K-12 strain W3110 using the Expand High Fidelity PCR System (Roche) and the primers JG1 and JG2. The 1.05-kb Ag43 PCR product was digested with EcoRI/HindIII, then ligated into pBAD24 vector digested with EcoRI/HindIII to generate pBAD24::Ag43. Using the primers DR5, DR6 and pBAD24::Ag43 as template, a PCR product encoding the Ag43 gene was amplified, digested with EcoRI/HindIII and ligated into pTrc99a digested with EcoRI/HindIII to construct the plasmid pTrc99a::Ag43. This plasmid was then used as a template for site-directed mutagenesis PCR using the primers DR7 and DR8 to introduce the mutation D551N constructing pTrc99a::Ag43(D551N), which in turn was used as a template to construct the His-tag derivatives pTrc99a::His-Ag43(D551N) and pTrc99a::Ag43(D551N)-His. To construct pTrc99a::Ag43(D551N)-His, a PCR product encoding a C-terminal His-tag of Ag43(D551N) was produced by use of the primers DR9 and DR10, digested with EcoRI/HindIII and ligated into pTrc99a digested with EcoRI/HindIII. The N-terminal His-tag derivative pTrc99a::His-Ag43(D551N) was constructed by PCR using the primers DR11 and DR12 that introduced a His-tag behind the 50 amino-acid signal sequence of Ag43. To mutate T878 to a stop codon-constructing Ag43(T878), a mutagenesis PCR was performed using primers DR17 and DR18 and pTrc99a::Ag43(D551N) as a template. The α 43 -domain-encoding part of the flu gene including the signal peptide of Ag43 was amplified using pTrc99a::Ag43 as a template and the primers DR13 and DR14, digested with EcoRI/HindIII and ligated into pTrc99a that had been digested with EcoRI/HindIII to construct pTrc99a::α 43 . Since the β 43 -domain contains no signal peptide of its own, it was amplified using pTrc99a::Ag43(D551N)-His as a template and the phosphorylated primers DR15 and DR16 to gain a blunt-ended β 43 -encoding PCR fragment that was ligated directly into the pTrc99a derivative coding for an OmpA signal peptide as described for the construction of pTrc99a::OmpA sp /HpmA*126. The bamA – E genes were amplified by PCR from genomic DNA isolated from E. coli DH5α cells. BamA was amplified using the primers O58 and O59, bamB with the primers O56 and O124, bamC with the primers O66 and O67, bamD with the primers O68 and O69 and bamE with the primers O71 and O129. Finally, the bamA PCR product was digested with NdeI/AatII and the bamB product with NcoI/NotI. Both were ligated together into a pETDuet vector (Novagen) digested with NdeI/NotI to construct the plasmid pAHB90 containing a Strep tag at the C-terminal end of BamB. The bamC PCR product was digested with NcoI/NotI and the bamD product with NdeI/AatII. Both were ligated together into a pACYduet vector (Novagen) digested with NdeI/NotI to construct the plasmid pAHB46. The bamE PCR product was digested with NcoI/XhoI and ligated into pET24d vector (Novagen) digested with NcoI/XhoI to construct the plasmid pAHB85 with a C-terminal His-tag on BamE. Reconstitution of proteoliposomes The isolation of outer membranes was performed as described with slight modifications [19] , [45] . Briefly, after 3 h growth at 37 °C, cells of wild-type strain BL21(DE3) or BL21(DE3) cells overexpressing the Isopropyl β- D -1-thiogalactopyranoside (IPTG)-induced transporters FhaC or ShlB were collected by centrifugation (8,650 g ), washed once and disrupted in a French Press. A crude membrane fraction was collected from the cell extracts by centrifugation at 150,000 g for 2 h at 4 °C. Finally, the outer membranes were isolated by sucrose gradient centrifugation at 82,000 g for 17 h at 4 °C in a Sorvall AH-629 swing-out rotor. The sucrose gradient was composed of 9 ml of 0.77 M, 16 ml of 1.44 M and 9 ml of 2.02 M sucrose. The outer membranes were collected from the lower interface, diluted sevenfold with 50 mM triethanolamine acetate (TeaOAc), pH 7.5, pelleted at 150,000 g for 2 h at 4 °C and resuspended in OMV buffer (50 mM TeaOAc, pH 7.5, 250 mM sucrose) to give an absorbance at 280 nm of 40 μ ml −1 , which was determined after diluting the suspension of outer membrane vesicles 100-fold in 2% SDS, aliquoted, frozen in liquid nitrogen and stored at −80 °C. Reconstitution of OMP proteoliposomes containing the pool of OMPs was performed as described [19] with modifications. Method 1: 20 μl of outer membranes from either wild-type cells or strains overexpressing the FhaC or ShlB proteins was solubilized by dilution into 400 μl of solution PE (20 mM Na 2 HPO 4 , 1% Elugent) and incubation at room temperature for 2 h by end-over-end rotation. Following an ultracentrifugation at 100,000 g for 1 h at 4 °C to remove insoluble material, the supernatant was mixed with 300 μl of 20 mM Na 2 HPO 4 and 200 μl of solution PE containing 2 μg μl −1 Avanti E. coli phospholipids. A 50 μg μl −1 stock solution of phospholipids was prepared by suspending the dried powder in water and sonicating overnight at 4 °C. The stock solution was applied to several freeze/thaw cycles before use. The OMP-phospholipid mixture was added to a SafeSeal Microcentrifuge tube (BioScience) containing 50–65 mg Biobeads SM-2 Adsorbent, 20–50 mesh (Bio-Rad). The Biobeads had been pretreated by washing them two times each with methanol, ethanol, double-distilled water and 20 mM Na 2 HPO 4 . The mixture was incubated for 2 h at 4 °C by end-over-end rotation, spun for 2 min at 16,000 g in a tabletop centrifuge and the supernatant was treated in the same manner for two more times with fresh batches of Biobeads with one rotation step being performed overnight. The proteoliposomes were recovered from the final supernatant by ultracentrifugation at 186,000 g for 30 min, and resuspended in 100 μl of OMV buffer. For the preparation of ShlB/FhaC proteoliposomes and BamA–E proteoliposomes, 0.72 μg of ShlB and 1.5 μg of purified BAM complex, respectively, were diluted with solution PE to give a final volume of 400 μl and used for reconstitution as described above. Method 2: for the experiments shown in Fig. 4 , 100 μl of outer membranes were mixed with 1.5 ml solution PE. OMPs were solubilized as described in method 1 and freed from insoluble material by centrifugation at 186,000 g for 30 min at 4 °C. The supernatant was divided into 200, 400 and 800 μl aliquots (corresponding to 1 × , 2 × , 4 × as indicated in Fig. 4 ). The volume of each tube was adjusted to 900 μl with solution PE and mixed with 200 μl of solution E containing 2 μg μl −1 phospholipids before reconstitution. All further steps were carried out as described for method 1. Protein purification For ShlB and FhaC purification, a 12-fold amount of solubilized and cleared outer membrane extract (240 μl membranes in 5 ml solution E, prepared according to method 1) containing overexpressed ShlB or FhaC was transferred to an Amicon Ultra-4 Centrifugal Filter Unit and centrifuged at 4,400 g until concentrated down to 1 ml. Fifty μl was collected for SDS–PAGE analysis as in Fig. 1c (Load). For batch purification, a gravity flow column was prepared from 1.5 ml of a 50% slurry of Talon beads (Clontech). The Talon beads were first equilibrated with 2 ml solution PE, then loaded with 1 ml of concentrated outer membrane extract. The flow through was collected and 50 μl was removed for analysis as in Fig. 1c flow through (FT). The column was washed three times with 1 ml each of solution PE containing 5 mM imidazol. Bound ShlB or FhaC was eluted by applying three times 1 ml each of solution PE containing 200 mM imidazol. The wash and elution fractions were collected and 50 μl of each sample was analysed by SDS–PAGE ( Fig. 1c ). For the co-expression of all BAM subunits (BamA–E), BL21(DE3) cells were transformed with plasmids pAHB90, pAHB46 and pAHB85 and grown in luria broth (LB) medium at 37 °C to an OD 600 of ~0.6. Expression was induced by the addition of 0.1 mM IPTG and the temperature was shifted to 18 °C. After 4 h, cells were harvested by centrifugation and pellets were dissolved in 20 mM Tris–HCl, pH 8.0. Cells were broken using a Constant cell disruption system (Constant Systems) at a pressure of 2.2 bar. Remaining cells were removed by centrifugation at 13,000 g and membranes were collected by ultracentrifugation at 200,000 g for 30 min. To extract proteins, the collected membranes were homogenized in 1 × Tris-buffered saline (TBS; 50 mM Tris/HCl, pH 7.5, 150 mM NaCl) containing 1% DDM ( n -dodecyl- D -maltoside) for 1 h. Non-solubilized material was removed by ultracentrifugation at 200,000 g for 30 min. The cleared membrane extracts were applied to a Strep-Tactin affinity column and proteins were eluted with 1 × TBS containing 0.02% DDM and 2.5 mM desthiobiotin. The BAM complex was further purified by size-exclusion chromatography using a 10/300 or PC 3.2/30 Superose 6 column equilibrated with 1 × TBS containing 0.02% DDM. Protein translocation and integration assay Spheroplasts were prepared from E. coli BL21(DE3) cells that had been transformed with the desired plasmids and grown overnight in 5 ml of minimal E-medium (2 mg ml −1 citric acid·1H 2 O, 0.2 mg ml −1 MgSO 4 ·7H 2 O, 13.1 mg ml −1 K 2 HPO 4 ·3H 2 O, 3.5 mg ml −1 NaNH 4 HPO 4 ·4H 2 O, 0.4% glucose, 100 μM of each proteinogenic amino acid, except methionine and cysteine) supplemented with appropriate antibiotics. The cells were pelleted at 4,400 g , resuspended in TS buffer (100 mM Tris/HCl, pH 7.5, 0.5 M sucrose) to achieve a final OD 580 of 4 and combined with an equal amount of LE buffer (0.1 mg ml −1 lysozyme, 8 mM EDTA, pH 8.0), then incubated on ice for 15 min. Spheroplasts were harvested by spinning at 4,400 g at 4 °C for 15 min and were resuspended in E-medium, in which glucose was replaced by 2% glycerol and 0.25 M sucrose to achieve a final OD 580 of 4. Spheroplasts secreting individual proteins were adjusted to a final OD 580 of 8 (β 43 ), 0.08 (α 43 ), 0.2 (FhaB*37), 0.8 (HpmA*126, Ag43(D551N) derivatives, BamA and OmpA) and 0.002 (Ag43(T878)). The translocation experiments were performed in a co-secretional manner, in which the spheroplasts were first incubated at 37 °C for 15 min, then induced with 4 mM IPTG for protein expression followed by another 3 min incubation before adding 8 μl ml −1 [ 35 S]-EasyTag Express Protein Labeling Mix. Spheroplasts (110 μl) were then immediately mixed with 1 μl liposomes/OMP proteoliposomes or 10 μl of ShlB/FhaC proteoliposomes or BAM proteoliposomes (for Ag43) and incubated for another 15 min at 37 °C for protein translocation experiments. After removing the spheroplasts by low-speed centrifugation at 13,000 r.p.m. for 6 min, the supernatant was divided into two halves: one half was precipitated directly with trichloroacetic acid (TCA; 5% final concentration), while the other half was treated with 500 μg ml −1 PK for 25 min at 25 °C followed by addition of TCA (5% final), incubation at 56 °C for 10 min to inactivate PK and transfer of the sample onto ice for precipitation. The pellet was collected in a tabletop centrifuge at 16,000 g for 10 min and after removal of the supernatant dissolved by heating at 95 °C in 15 μl Laemmli sample buffer for 5 min. Translocation efficiencies were calculated from the ratio of PK-resistant bands versus non-treated species using ImageQuant 5.2 (GE Healthcare). The integration assays were performed in a post-secretional manner, in which spheroplasts were first removed by centrifugation after 3 min pulse labelling and 110 μl of separated supernatants was each mixed with 2 μl of liposomes or proteoliposomes and incubated for 15 min at 37 °C. After integration, the reaction mixture was divided into two aliquots. For integration assays of OmpA, both aliquots were directly subjected to TCA precipitation and finally dissolved in Laemmli sample buffer. One aliquot was heated at 95 °C for 5 min, while the other aliquot was incubated at 37 °C for 15 min, both under shaking with 14,000 r.p.m. For integration assays of BamA, the TCA precipitation was omitted and both aliquots were directly mixed with 5 × Semi-SDS loading buffer (0.665 M Tris/HCl, pH 6.8; 50 mM EDTA, pH 8.0; 5% SDS; 50% glycerol; 0.25% bromophenol blue), then one aliquot was heated at 95 °C for 5 min with shaking at 14,000 r.p.m. while the other aliquot was not further treated. All BamA samples were loaded on 10% polyacrylamide gels containing no SDS, and electrophoresis was performed at 4 °C overnight. Integration efficiencies were calculated from the ratio of folded species versus the sum of folded and unfolded species using ImageQuant 5.2 (GE Healthcare). For the experiments depicted in Fig. 4 , spheroplasts from E. coli BL21(DE3) cells transformed with pTrc99a::FhaC or empty pTrc99a were generated and 100 μM each of cold methionine and cysteine were added during a mock labelling period. In this case, 1 ml spheroplasts was mixed with 100 μl of reconstituted OMP or BAM proteoliposomes and incubated for 60 min at 37 °C to allow for the integration of FhaC. The spheroplasts were then removed by centrifugation at 17,000 g in a tabletop centrifuge for 6 min. The supernatant was subsequently subjected to ultracentrifugation at 186,000 g for 30 min at 4 °C to pellet OMP or BAM proteoliposomes, which were resuspended in 100 μl OMV buffer. These OMP or BAM proteoliposomes (8 μl per reaction) were used immediately for FhaB*37 translocation experiments as described above. Western blot Detection of FhaC and its mutants by western blot was performed using 10 μl of proteoliposomes each and standard SDS gels. For detecting BamA by western blotting, 5 μl outer membranes (OD 280 =35 μ ml −1 ) isolated from BL21(DE3) strain was mixed with 25 μl 1 × semi-native SDS-loading buffer, then loaded on 10% polyacrylamide gels containing no SDS and electrophoresis was performed overnight at 4 °C. Afterwards, the proteins were transferred onto a nitrocellulose membrane, which was then blocked overnight in phosphate-buffered saline (PBS; 140 mM NaCl, 2.7 mM KCl, 10 mM Na 2 HPO 4 ·2H 2 O, 2 mM K 2 HPO 4 , pH 7.6) containing 5% non-fat dried milk, and incubated with anti-BamA antibodies [46] (1:10,000 dilution). The blot was washed with PBST (PBS containing 0.15% Tween-20) and developed with ECL Western Blotting Detection Reagents (Amersham), then detected with Fusion Fx7 (PEQLAB Biotechnologie GmbH). Original images of all western blots are shown in Supplementary Figs 1–3 . Flotation experiments For flotation analysis, a three-layered discontinuous sucrose gradient was generated within a 1-ml Thickwall polycarbonate centrifugation tube (Beckamn Coulter). A mixture of 100 μl of OMP proteoliposomes containing de novo integrated FhaC and 100 μl of 2.5 M sucrose was overlaid with 500 μl flotation buffer (50 mM TeaOAc, pH 7.5, 8 mM MgAc, 70 mM KAc, 1 mM DTT) containing 1 M sucrose followed by a top layer that consisted of 300 μl flotation buffer. After centrifugation in a Sorvall S100-AT4 rotor at 540,628 g for 90 min, four 250 μl fractions were carefully collected from top to bottom and transferred into separate tubes. Any remaining pellet was dissolved by adding 25 μl Laemmli sample buffer and boiling for 5 min. The top three fractions were combined and then precipitated with TCA (7.5% final). The fourth fraction was separately precipitated with TCA. Finally, the pellets were dissolved in Laemmli sample buffer and separated on 10% SDS–PAGE, which was developed by western blotting using antibodies against FhaC (ref. 20 , used at 1:5,000 dilution). Quantification of the bands was performed with ImageQuant 5.2 (GE Healthcare). How to cite this article: Norell, D. et al . Versatile in vitro system to study translocation and functional integration of bacterial outer membrane proteins. Nat. Commun. 5:5396 doi: 10.1038/ncomms6396 (2014).